A novel methodology for large-scale phylogeny partition The spread of type-1 human immunodeficiency virus (HIV-1) infection is influenced by a long duration of the asymptomatic stage, a high viral evolutionary and replication rate, as well as population movements, social behaviour and geopolitical factors such as infrastructure development and accessibility [1] , [2] . Phylogenetic analysis can be used to investigate HIV-1 transmission events, although the long period of infectivity, coupled with often non-uniform spatial and temporal sampling, can limit its efficiency in tracing the infection chains [3] , [4] , [5] . Several epidemiological factors, for example the mode of HIV-1 transmission or the disease stage, might be associated to different transmission lineages. Antiretroviral therapy (ART) usually suppresses HIV-1 replication, reducing the probability of virus transmission [6] , [7] , [8] . Drug-resistant strains can be selected by ART exposure, and transmitted from patients failing ART or from drug-naive patients already carrying a drug-resistant virus [9] , [10] . Given the decreasing prevalence of virological failures among HIV-1-infected patients and of viraemic patients carrying drug resistance over time [11] , a greater proportion of transmitted resistance may be derived from ART-naive subjects [12] , [13] , [14] . Transmission clusters among HIV-1-infected patients have been inferred and analysed across various study cohorts, including the United Kingdom [15] , [16] , [17] , [18] , Switzerland [19] , [20] , Canada [21] and the Netherlands [22] . Nowadays, parallel computation techniques permit the estimation of highly resolved phylogenies for large populations [20] . However, the partition of phylogenetic trees [23] , [24] is a challenging task and there is not yet an established automated consensus methodology to identify transmission clusters, particularly when considering large-scale phylogenies. Furthermore, the definition of a transmission cluster itself is not standardized [15] , [16] , [17] , [18] , [19] , [20] , [21] , [22] . Transmission clusters have been associated to sub-trees of phylogenies containing sequences from at least x distinct subjects [15] , [16] , [17] , [18] , [19] , [20] , [21] , [22] (from a minimum of two patients to more than ten patients) with a sub-tree reliability of ≥ y % (usually bootstrap support or posterior probability, ranging from 80 to 99% [21] , [18] ). Geographical constraints, that is, ≥ z % of sequences from the same country in a cluster (usually z ≥ 80%), have been also introduced [20] . Often, unrelated viral strains from different countries are added as controls, and clusters are identified by visually inspecting an initial tree or by re-estimating smaller trees after reducing the original data set [15] , [17] . Cluster selection based on absolute genetic [15] , [17] and patristic [18] , [21] distance values has also been used. This work proposes a new approach for the automated partition of large phylogenies, by introducing a flexible (yet statistically robust) definition of a transmission cluster, which fits also the previously introduced definitions. The method is then applied for identifying transmission clusters within the HIV-1 subtype B epidemic in Italy. Data were drawn from the Antiretroviral Resistance Cohort Analysis (ARCA), a national observational cohort of HIV-1-infected patients ( http://www.hivarca.net ) followed up at 105 clinical centres. At the time of this study, data from >20,000 patients and >23,000 HIV-1 pol gene sequences were available. A phylogeny on the Italian HIV-1 subtype B isolates was estimated by parallel computation and, after applying the new partition method, clustering was linked with patients' demographic and clinical information. As a result, several factors associated with transmission chains were identified, suggesting strategies to monitor the epidemic. The methodology proposed here provides a general and robust framework for analysing large-scale phylogenies that can be applied in investigating the molecular epidemiology and the intra-host evolutionary patterns of a broad range of pathogens. Automated partition of phylogenetic trees The definition of transmission cluster introduced here requires a rooted phylogeny and assumes that two or more patients belong to a potential transmission cluster if their viral sequences are monophyletic and more closely related than those from two randomly selected individuals. The meaning of 'more closely related' refers to the comparison with a distance threshold formally defined as follows. Given a rooted phylogeny, the distribution of all patristic distances between pairs of taxa (whole-tree distribution) and the distribution of all pairwise patristic distances within any sub-tree (sub-tree distribution) are defined. Then, a specific sub-tree is classified as a transmission cluster if the median value of its distance distribution is below a t -percentile threshold (which needs to be properly tuned, see below) of the whole-tree distribution. As complimentary constraints, a sub-tree is considered to be eligible as transmission cluster only if it contains sequences from ≥2 subjects and has a reliability ≥90%. It is important to notice that both the threshold (either t -percentile of the whole-tree distribution or a specific cutoff value) and the other constraints can easily be modified so that they conform to previously introduced definitions. To extract clusters from a phylogeny, a depth-first algorithm was used, which is a general strategy for traversing a graph or a tree. In brief, after calculating the whole-tree distance distribution, the depth-first ( Fig. 1 ) starts from a root node and moves into a sub-tree, checking its reliability, number of leaves and calculating the sub-tree distribution. If the clustering conditions are not met, the algorithm goes deeper into another child sub-tree, otherwise it stops, and the leaves of the current sub-tree are placed in a cluster. Then the search restarts from the most recent sub-tree that has not been visited. If a leaf is reached, no clusters are identified for that path. 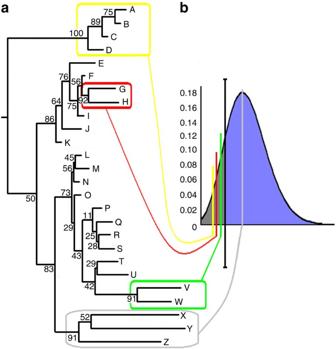Figure 1: Automated partition of a phylogenetic tree. Graphical example of a depth-first tree search for automated phylogenetic tree partition. The method considers nodes/sub-trees with a reliability ≥ 90% and ≥ 2 distinct patients, recognizing a sub-tree as a cluster when the median sub-tree pairwise patristic distance is below a percentile threshold of the whole-tree patristic distance distribution (let it be the 10th percentile). (a) An example of a phylogenetic tree, where each patient/sequence is identified by a letter (A–Z) and each tree node has an associated value of reliability (which might be bootstrap support). (b) Histogram of the whole-tree patristic distance distribution. The vertical black line corresponds to the 10th percentile distance threshold. The partition method identifies three clusters (yellow, red and green) and discards the grey sub-tree. Figure 1: Automated partition of a phylogenetic tree. Graphical example of a depth-first tree search for automated phylogenetic tree partition. The method considers nodes/sub-trees with a reliability ≥ 90% and ≥ 2 distinct patients, recognizing a sub-tree as a cluster when the median sub-tree pairwise patristic distance is below a percentile threshold of the whole-tree patristic distance distribution (let it be the 10th percentile). ( a ) An example of a phylogenetic tree, where each patient/sequence is identified by a letter (A–Z) and each tree node has an associated value of reliability (which might be bootstrap support). ( b ) Histogram of the whole-tree patristic distance distribution. The vertical black line corresponds to the 10th percentile distance threshold. The partition method identifies three clusters (yellow, red and green) and discards the grey sub-tree. Full size image To analyse the effect of the threshold t , two independent data sets of different sample sizes ( n =127 and n =1,204 sequences) were used, comprising HIV-1 subtype B pol sequences obtained either from patients belonging to epidemiologically confirmed transmission clusters (plus a set of control sequences) or by visually selecting the transmission chains from the phylogenetic tree. Our method yielded rates of agreement with the epidemiologically confirmed/visually determined transmission events up to 93%. The optimal threshold interval ranged from the 10th to the 35th percentile, with a corresponding absolute distance range of 0.04–0.08 nucleotide substitutions per site ( Supplementary Fig. S1 ). Additional sensitivity analyses were conducted by comparing cluster sizes, cluster numbers, distance and branch length distribution of the study and the validation sets, and by comparing against randomly generated trees (Methods). Application of the partition method to HIV-1 phylogeny A total of 11,541 HIV-1 subtype B pol sequences from 7,350 patients were included in the analysis, plus two outgroups (subtype C and J). Multiple sequence alignment and maximum-likelihood phylogeny, excluding drug-resistance mutation sites, were carried out using parallel computation. 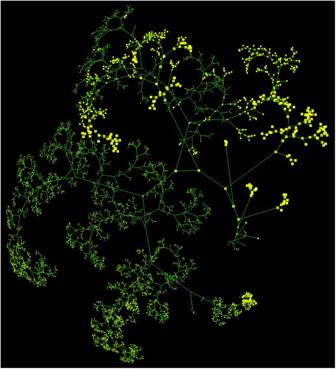Figure 2: Phylogeny of Italian HIV-1 subtype Bpolisolates. Maximum-likelihood phylogenetic tree of 11,541 HIV-1 subtype Bpolgene sequences from the Italian ARCA cohort. Tree is rooted on subtype J and depicted using three-dimensional hyperbolic geometry. Nodes and leaves are highlighted by yellow points. 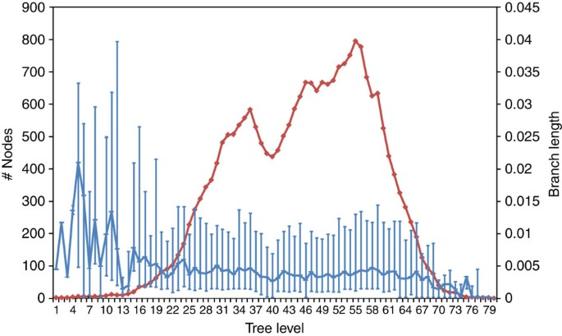Figure 3: Tree topology. Topological analysis of a maximum-likelihood phylogenetic tree composed of 11,541 HIV-1 subtype Bpolsequences from the Italian ARCA cohort, rooted on subtype J. Median (interquartile range) branch length (blue) and number of nodes (red) for each tree level are depicted. Figure 2 shows the phylogenetic tree, whereas Figure 3 depicts the median and interquartile (IQR) values of branch lengths from a parent node to the child and of number of nodes across the tree levels, starting from the root. Branch lengths and node levels showed a minimal inverse correlation ( r =−0.023, P <0.0001). There was also a low but statistically significant correlation between the calendar dates of the leaves and the root-to-tip distances ( r =0.25, P <0.0001, Supplementary Fig. S2 ), confirmed on a multivariable analysis ( Supplementary Table S1 ). Figure 2: Phylogeny of Italian HIV-1 subtype B pol isolates. Maximum-likelihood phylogenetic tree of 11,541 HIV-1 subtype B pol gene sequences from the Italian ARCA cohort. Tree is rooted on subtype J and depicted using three-dimensional hyperbolic geometry. Nodes and leaves are highlighted by yellow points. Full size image Figure 3: Tree topology. Topological analysis of a maximum-likelihood phylogenetic tree composed of 11,541 HIV-1 subtype B pol sequences from the Italian ARCA cohort, rooted on subtype J. Median (interquartile range) branch length (blue) and number of nodes (red) for each tree level are depicted. Full size image By applying our partition method, the number of clusters retrieved using three distinct absolute distance thresholds of 0.04, 0.07 and 0.08 nucleotide substitutions per site (corresponding to the 1st, 15th and 30th percentile thresholds) were 842, 587 and 292, respectively. For each threshold, each cluster had a median (IQR) number of 3 (2–6), 4 (2–9), and 4 (2–10) distinct patients, respectively ( Supplementary Fig. S3 ). The proportion of clustered isolates was 41.71, 73.44 and 92.23%. Of note, at the 30th percentile threshold, about a half of the sequences were placed in two distinct clusters ( n =5,785 and n =1,538), both exceeding in size the number of un-clustered isolates ( n =897). At thresholds below the 30th percentile, the maximum cluster size was always inferior to the number of un-clustered isolates ( Supplementary Fig. S4 ). Thus, the 30th percentile threshold behaved as a break-point: all subsequent analyses yielded similar results across lower thresholds, whereas the same did not always held when considering both thresholds above and below the break-point. The partitions retrieved at different thresholds exhibited a mild rate of agreement, with a peak at the 15th percentile threshold ( Supplementary Fig. S5 ). Notably, two previously published cases [25] , [26] of drug-resistance transmission from ART-naive to ART-naive patients in ARCA were correctly identified at any of the thresholds considered. Transmission clusters and factors associated with clustering The phylogeny partition was linked to the patients' epidemiological and clinical information. Descriptive statistics of the study population is shown in Table 1 . Table 1 Study population. Full size table Table 2 describes the composition of clusters when considering the threshold distance of 0.07 (15th percentile, highest rate of agreement). Sequences without epidemiological information were ignored, and only the earliest available sequence per patient was considered. Each cluster was evaluated checking if it was composed exclusively either by a single or by a mixture of different demographic factors. The estimated proportions were then compared against those that would be expected by chance after randomly shuffling the cluster indices. We found an excess in the proportion of clusters composed solely by patients living in the Northern Italy (31 versus 17%, P <0.0001), by those living in the Central Italy (25 versus 16%, P =0.0008), by male homosexuals (27 versus 16%, P <0.0001), by male homosexuals and heterosexuals together (20 versus 10%, P <0.0001), by patients infected recently (within three years from the first HIV-1 positive test, 35 versus 19%, P <0.0001), by ART-naive patients without any drug-resistance mutation (15 versus 6%, P <0.0001), by patients with high HIV-1 RNA load (above 10,000 copies per ml, 43 versus 34%, P =0.02), by patients carrying at least one resistance mutation to nucleoside/nucleotide reverse transcriptase inhibitors (NRTI) and protease inhibitors (PI) (26 versus 19%, P =0.007; 10 versus 6%, P =0.02, respectively). Conversely, we observed a proportion significantly lower than expected for clusters comprising male homosexuals and injecting drug users (IDUs) together (3 versus 9%, P <0.0001), male homosexuals and heterosexuals and IDU together (11 versus 25%, P <0.0001), and patients living in the Northern Italy and in the Central Italy (27 versus 42%, P <0.0001). Notably, although the proportions of clusters composed by patients either naive or carrying any drug-resistance mutation were exceeding those expected by chance, along with the mixtures of ART-exposed/ART-naive and patients with/without resistance, there was no excess in the proportion of naive patients carrying any drug-resistance mutation (2 versus 2%, P =0.898). Similar results were obtained by considering thresholds up to the 30th percentile (data not shown). Table 2 Demographic factors in transmission clusters. Full size table In Table 3 , we report the results from a multivariable analysis conducted calculating the odds of being/not-being included in a transmission cluster, for the thresholds at the 1st, 15th and 30th percentile. At any of the thresholds considered, a higher HIV-1 RNA and a higher CD4+ count were associated with clustering, along with a more recent infection and a younger age. On the contrary, the presence of at least one drug-resistance mutation to NRTI and PI was not associated with clustering. The mode of HIV transmission was the factor that exhibited opposite behaviours by varying the threshold: at low thresholds male homosexuals and heterosexuals tended to cluster more than IDU, whereas the contrary held at higher thresholds. This might be explained by the fact that IDU have a larger pool of contacts as compared with homosexuals/heterosexuals and thus are more likely to be included in larger transmission chains characterized by greater genetic diversity [27] . Table 3 Factors associated with transmission clustering. Full size table A new methodology for the partition of large-scale phylogenies and the inference of transmission clusters was introduced. This approach conjugates the evaluation of node reliability, tree topology and patristic distance analysis. Previous approaches have lacked, in general, not only a standardized definition of a transmission cluster, but also a formal algorithmic procedure for the detection of reliable transmission clusters within a phylogeny. In the studies by Lewis et al . [15] and Hughes et al ., [17] clusters were identified on large data sets using a fixed threshold on genetic distances, and then confirmed by phylogenetic trees constructed afterwards. Another approach was the CTree algorithm [24] , originally applied to viral sub-typing, which does not account for node reliability and is not applicable to large data sets in its current implementation. Other available methods have used different cluster selection schemes by performing nested phylogenetic analyses, and/or adding criteria for geographical consistency [15] , [16] , [17] , [18] , [19] , [20] , [21] , [22] , but in most cases the assessment of transmission clusters is still subject to a visual tree inspection. The definition of a transmission cluster proposed here is general and can be tuned to accommodate any of the previous definitions. The method can be of interest for epidemiologists because obtained partitions could be used in multi-level modelling. The depth-first approach was applied to a large study population, composed of viral sequences of HIV-1-infected patients followed up at the Italian clinics, with the aim to gain knowledge about viral transmission clusters and their associated factors. The transmission clusters detected in our study population were preferentially composed either by male homosexuals only or by male homosexuals and heterosexuals together. As male homosexuals (and presumably male bisexuals) are a primary source of the cluster composition, this could be considered for designing targeted population screenings and interventions. On the other hand, there was a negative association between male homosexuals/heterosexuals and IDU. We found that ART-naive patients cluster both with other ART-naive and with ART-experienced patients, in various configurations with respect to the carriage of drug-resistance mutation. Although the direction of the transmission cannot easily be inferred, the proportion of clusters composed exclusively by ART-naive patients carrying at least one drug-resistance mutation in our population study (so presumably transmitting the resistance to each other) was ≈2%, a low proportion, comparable to a previous estimation in the United Kingdom [16] . A substantial responsibility of drug-resistance transmission is still carried by the ART-experienced population, suggesting that any decrease in the prevalence of drug-resistance in the ART-experienced population could translate into a reduction of the proportion of new infections with drug-resistant virus. Multivariable analysis revealed several factors independently associated with the transmission clustering, including a higher HIV-1 RNA load and CD4+ count, but not the presence of drug-resistance. These results partially agree with those reported from the Swiss cohort study [19] , in which the strongest predictor of clustering was the detection of drug-resistance, along with HIV-1 RNA load and CD4+ count. However, that study population was composed by newly diagnosed individuals. The association of a recent HIV-1 positive test with transmission clustering could be simply due to the fact that in these individuals the intra-host viral evolution is at an early stage and thus it is easier to trace the possible transmission source. Another possibility, however, is that some newly infected patients might not be aware of being infected, and therefore continue to engage in risky sexual behaviours. Recently, infected and untreated patients are also more likely to have higher viral loads, resulting in higher probability of transmission [6] . Thus, efforts to expand HIV-1 testing programmes should be a successful strategy to reduce the rates of HIV-1 transmission. Concomitantly, the association of higher HIV-1 RNA loads and CD4+ counts with transmission clustering emphasizes the need of early diagnoses and suggests how early treatment may be useful in reducing HIV-1 transmission events. This work has some limitations. First, epidemiological conclusions may change slightly or dramatically depending on the choice of the threshold. By evaluating the algorithm on different data sets, and using different definitions of a transmission cluster, the optimal threshold spanned a large range, from 0.04 to 0.08 nucleotide substitutions per site, whereas previous studies used more stringent criteria (either 0.015 or 0.031) [18] , [21] . Ideally, a transmission chain, at least in the context of a single subtype phylogeny of HIV-1 isolates, should be defined by an absolute threshold. At the moment, the lack of epidemiologically confirmed data precludes such a precise estimation. Nonetheless, the present method offers a rational validation strategy to identify an appropriate cutoff, depending on the specific data set under investigation and on the (strict or loose) definition of a transmission cluster. Second, complete demographic and clinical information were missing for a relevant proportion of patients enrolled in ARCA. A non-uniform sequence sampling has most likely occurred overtime. Most of the sequences included in our analysis were derived from ART-experienced patients tested at virological failure. Although repeated measures and convergent evolution due to treatments were accounted for, the analysis lacked a sample contribution from recently infected patients. Sampling could potentially distort results when analysing factors associated with transmission chains [20] . Finally, the partition method is fully dependent on the phylogenetic tree: if the tree is unreliable, then so is the cluster identification. The estimation of highly resolved and reliable phylogenies from large data sets is still a challenge and requires massively parallelized routines, especially for maximum likelihood or Bayesian tree inference. For this reason, the approach based on nested phylogenies might be still a preferable choice. Some limitations of phylogenetic efficiency in detecting transmission chains [3] could also be overcome by coupling phylogeny inference with models derived from the complex network theory [28] , [29] , [30] , [31] . For instance, a phylogeny could be used as a previous knowledge to infer sexual links when designing a social network model for HIV-1 infection. The analysis of transmission clusters using the method discussed herein can easily be extended to non-B subtype HIV-1, whose circulation is increasing in the Italy and Europe [32] , as well as other viral epidemics, such as hepatitis B or C viruses (HBV/HCV), influenza and coronavirus infection. In particular, HCV is one of the fastest growing pandemics and its evolutionary rate, genetic heterogeneity and risk transmission factors are similar to HIV-1. Given the upcoming availability of HCV antivirals, surveillance of drug-resistance and analysis of transmission clusters using standardized algorithms are expected to be of outstanding interest in the near future. Finally, the algorithm described here can potentially be used in the study of intra-host phylogenies—especially for the characterization of infected cellular reservoirs and compartments in viruses such as HIV [33] , [34] , [35] , [36] or simian immunodeficiency virus [37] —in terms of viral fitness, emergence of drug resistance and pathogenesis. Study population HIV-1 pol gene sequences (encompassing at least amino acidic positions 1–99 of protease and 1–250 of reverse transcriptase) of ART-naive and ART-experienced patients were extracted from ARCA, with sampling dates, plus corresponding information (where available) on patients' age, gender, country of origin, country area of residence, mode of HIV-1 transmission, date of first HIV-1-positive test, date of first ART, HIV-1 RNA load and CD4+ T cell count contemporary to the sampling date (between −30/+7 days for HIV-1 RNA, between −30/+30 days for CD4+). Sequence analysis Viral subtype was assigned by using the Rega subtyping tool ( http://www.bioafrica.net/rega-genotype/html/subtypinghiv.html ). All sequences classified as subtype B, excluding any putative recombinant form, were aligned using the parallel implementation of ClustalW [38] , and manually edited. Resistance to an antiretroviral class (nucleoside-tide/non-nucleoside/protease inhibitors) was defined as the presence of at least one major mutation conferring resistance to at least one drug belonging to that class according to the 2009 update of the International AIDS Society reference list ( http://www.iasusa.org/resistance_mutations/mutations_figures.pdf ). Deduced amino-acid mixtures including a major resistance mutation were considered as indicative of resistance, unless otherwise specified. Columns of the multiple alignment corresponding to codon positions associated to drug-resistance were removed. Phylogenetic analysis Maximum-likelihood phylogenetic analysis was performed on the alignment, adding HIV-1 subtypes J and C as outgroups. The parallel implementation of FastTree software [39] was used, setting up a general-time-reversible model, with a 20-parameter gamma optimization, and a mix of nearest-neighbour interchanges and sub-tree/prune/regraft moves for tree topology search. Reliability of each tree split was calculated by a Shimodaira–Hasegawa test. To visualize the large tree as a whole, three-dimensional hyperbolic geometry software was used ( http://www.caida.org/tools/visualization/walrus/ ). Parallel ClustalW multiple alignment required ∼ 10 h on a two quad-core 64bit Intel Xeon X5550@2.66GHz, with Hyper-Threading technology, using a total of 16 processing units and 24GB DDR3 RAM. Parallel FastTree software run for ≈ 40 min. Automated partition of phylogenies After obtaining the maximum-likelihood phylogenetic tree, rooted on HIV-1 subtype J, tree topology was analysed with a depth-first visit [40] by considering the number of sub-trees with a node reliability ≥ 90%, and an associated number of leaves with at least two distinct patients. At each step of the depth-first visit, a sub-tree was identified as a cluster if the median value of the sub-tree distance distribution was below a t -percentile threshold of the whole-tree distance distribution. If this condition was met in a node, the search at that node was stopped, ignoring the children nodes, passing to analyse other node siblings. The threshold t was evaluated and optimized over the range [5th, 50th] percentile of the whole-tree distance distribution, with a step of 0.05. Cluster partitions were compared by using the adjusted Rand index [41] . Software implementation and computational complexity Software has been implemented using the java ( http://java.sun.com/ ) programming language, released as a free platform-independent standalone application, executable both from the command-line and with a graphical user interface (downloadable as a Supplementary Software 1 and 2 , see Supplementary Note 1 , Supplementary Data 1 and 2 , and Supplementary Fig. S6 ). The software requires a phylogenetic tree input file in newick format. Three different options are available: (i) threshold-based partition algorithm, specifying a threshold value and a maximum number of distance comparisons; (ii) topological analysis, with median (IQR) values for branch length, reliability and number of nodes at each tree level; (iii) patristic distance calculator. In the partition algorithm (i), the calculation of the branch length difference distribution for a tree with k leaves, requires k* ( k -1)/2 pairwise comparisons, corresponding to 66.6 million for the ARCA phylogenetic tree. In the worst case, the depth-first search may require a number of accesses to the distance matrix, which is cubic in the number of entries. However, the implemented software has an efficient indexing routine that permit the exact calculation of a whole-tree distance matrix even for huge trees, at a price of a high random access memory usage. If the java virtual machine is initialized with at least 8 Gb of RAM, it is possible to compute exactly a full matrix for a tree with ≈10,000 leaves. Our routine for patristic distance calculation was validated by comparing it against the 'cophenetic' function of the 'ape' library in the R software ( http://www.R-project.org ). Validation of partition method and threshold optimization The depth-first visit procedure for the automated partition of a phylogenetic tree was evaluated by using two different independent data sets. First, a maximum-likelihood phylogenetic tree was estimated (with the same alignment and tree fit procedures as previously described) by considering a set of group M subtype B HIV-1 pol sequences obtained from patients with a confirmed and known transmission history, plus a set of random control sequences from distinct patients of the same geographical area, and two outgroups (HIV-1 subtypes J and C). This data set was produced by querying the Los Alamos HIV repository ( http://www.hiv.lanl.gov/content/index ), in which 62 sequences from 35 patients were reported to be involved in five distinct transmission events. The number of control sequences was the same as that of sequences linked to the transmission events. Thus, a total of 127 sequences were considered in the subsequent phylogenetic analysis. The phylogenetic tree ( Supplementary Fig. S7 ) was also visually inspected to confirm the epidemiological evidence of transmission clustering, as follows. Identification of clusters was performed by examining leaves and nodes exhaustively. Only at a most recent common ancestor (MRCA) node with a reliability ≥ 90%, all the children leaves were iteratively grouped together, maximizing the cluster size, ensuring that any group included isolates from at least two distinct patients. In theory, if all nodes with a reliability of ≥ 90% were scored as transmission chains, then any highly supported epidemiological cluster with several nested highly supported transmission chains would also be considered as a transmission chain. However, if two potential transmission clusters happened to share a MRCA with a reliability value of ≥ 90%, but the two lineages departing from that MRCA exhibited long branch lengths, then they were considered as two independent transmission chains. Leaves that did not meet these criteria were left un-clustered. All transmission events were identified as distinct clusters, although some of the control sequences were placed in one or more of the five transmission clusters and additional clusters were identified ( n =12). The adjusted Rand index that compared the visual inspection of the phylogenetic tree against the epidemiological evidence was equal to 0.55. The depth-first procedure was executed optimizing the threshold t over a percentile interval range (5th, 50th) of the whole-tree distance distribution, with a step of 0.05, obtaining a maximum adjusted Rand index of 0.69 (11 clusters) at t =10th (0.04 nucleotide substitutions per site) percentile with respect to the epidemiological evidence and of 0.93 (10 clusters) at t =20th (0.062 nucleotide substitutions per site) percentile with respect to the visual clustering ( Supplementary Fig. S1 ). Successively, another maximum-likelihood phylogenetic tree was estimated on the whole set of group M subtype B HIV-1 pol sequences from the Los Alamos HIV repository, adding subtypes J and C as outgroups ( n =1,204), and transmission clusters were inferred by means of a visual inspection. The highest adjusted Rand index between the depth-first method and the visual inspection was 0.88, corresponding to a threshold of 0.08 nucleotide substitutions per site, that is, the 35th percentile ( Supplementary Fig. S1 ). As previously found [20] , the proportion of sequences that clustered together from the same country was significantly higher than expected by chance. We also compared the distributions of patristic distances and branch lengths in the validation sets and in the ARCA data set. Although significantly different in the sample size, the larger tree of Los Alamos ( n =1,204) and that of ARCA ( n =11,541) showed a remarkably low absolute difference in the average patristic distance values, which was below 0.004 nucleotide substitutions per site. The same held when considering the average branch length, with an absolute difference of 0.018 ( Supplementary Fig. S8 ). As a final evaluation, we compared the distributions of cluster number and cluster sizes across different percentile thresholds by considering several subtype B HIV-1 trees estimated on data sub-samples, against randomly generated trees (at different birth rates). At all thresholds below the 45th percentile, both the average number of clusters and the cluster size of real trees were significantly different from the values obtained by a random tree set ( Supplementary Figs S9 and S10 ). Epidemiological analysis Multivariable regression analysis was performed to identify prognostic factors of belonging to a transmission cluster (using a binomial link), and of root-to-tip distance (using linear regression). Generalized-estimating-equations models were used, using the 'geepack' library in the R software, with patient codes as identifiers. Covariate of interests were: sequence year (numeric), presence of for nucleoside-tide/non-nucleoside/protease inhibitor resistance mutations (binary), patient's area of residence (Northern/Southern/Central Italy or unknown), mode of HIV-1 transmission (heterosexual, male homosexual, IDU, other/unknown), gender (male/female/unknown), country of origin (Italian/non-Italian/unknown), age (categorized on the IQR range or unknown), ART status (ART-experienced/ART-naive/unknown), time passed from the first HIV-1 positive determination (categorized on the IQR range or unknown), HIV-1 RNA load and CD4+ cell count (numeric) at the time of genotyping. How to cite this article: Prosperi, M.C.F., et al . A novel methodology for large-scale phylogeny partition. Nat. Commun. 2:321 doi: 10.1038/ncomms1325 (2011).